Extreme diving behaviour in devil rays links surface waters and the deep ocean Ecological connections between surface waters and the deep ocean remain poorly studied despite the high biomass of fishes and squids residing at depths beyond the euphotic zone. These animals likely support pelagic food webs containing a suite of predators that include commercially important fishes and marine mammals. Here we deploy pop-up satellite archival transmitting tags on 15 Chilean devil rays ( Mobula tarapacana ) in the central North Atlantic Ocean, which provide movement patterns of individuals for up to 9 months. Devil rays were considered surface dwellers but our data reveal individuals descending at speeds up to 6.0 m s −1 to depths of almost 2,000 m and water temperatures <4 °C. The shape of the dive profiles suggests that the rays are foraging at these depths in deep scattering layers. Our results provide evidence of an important link between predators in the surface ocean and forage species occupying pelagic habitats below the euphotic zone in ocean ecosystems. Many marine predators dive regularly to forage on pelagic fish and squid populations in the deep ocean. Often concentrated in deep scattering layers (DSLs), these prey populations represent a significant, albeit largely unquantified, fraction of the earth’s aquatic biomass [1] . Large fish and mammals typically target prey within DSLs either by making repetitive feeding dives to mesopelagic depths of 400–800 m, or by following the same patterns of diel vertical migrations as those undertaken by many mesopelagic organisms [2] , [3] . Sperm whales ( Physeter macrocephalis ), for instance, regularly dive to mesopelagic depths where they are hypothesized to consume a biomass of squid equivalent to global marine landings on an annual basis [4] . Yet, very few species have been observed diving consistently beyond the mesopelagic into the bathypelagic zone, presumably because of physiological or energetic constraints that limit an animal’s ability to forage efficiently in environments characterized by high pressures, low temperatures and low levels of dissolved oxygen that are typically found at depths below 1,000 m. These constraints may prevent at least some ocean predators from accessing significant food resources in open oceans where maximum prey biomass can be located 1,000–2,500 m deep [5] . Deep-diving behaviour in marine fishes is often associated with physiological thermoregulatory capabilities that allow for the generation and retention of heat in critical tissues. Indeed, the convergent evolution of cranial endothermy in lamnid sharks and scombroid fishes suggests that the maintenance of brain activity and visual acuity in deep, cold waters has conveyed significant selective advantages to these groups over time [6] . While most endothermic fishes are apex predators, cranial endothermy has also been identified in several species of myliobatoid rays. For instance, several species of devil rays in the family Mobulidae possess well-developed retia mirabilia around the cranial cavity [7] . The presence of a heat-exchange system in these species was perplexing as mobulids were thought to be surface-dwelling filter feeders inhabiting warm temperate to tropical epipelagic waters. The authors concluded that the cranial rete cooled rather than warmed the brain as these rays were known to bask at the surface in tropical waters. More recent examinations [8] , [9] concluded that the retia in Mobula tarapacana and Manta birostris likely did act to warm the brain, although it was not clear what benefit the counter-current system provided for species that apparently did not encounter cold water. The difficulty assigning a function to retia mirabilia found in M. tarapacana highlights a lack of basic ecological information for pelagic mobulid rays. While members of the genus Mobula occur throughout tropical and warm-temperate oceans, we know little about horizontal or vertical movement patterns for any species. Two recent studies deployed satellite tags on Mobula japonica in the eastern north Pacific [10] and Mobula mobular in the Mediterranean Sea [11] . Tag data in both instances revealed relatively small horizontal and vertical movements in waters where temperatures were largely constrained between 20 and 30 °C. Neither study, therefore, provided information that might explain the presence of a counter-current heat exchange system in the genus. Here we report horizontal and vertical movements of M. tarapacana in the central North Atlantic Ocean. The results confirm that this species of devil ray is capable of traversing large distances through the oligotrophic open ocean. The data also document remarkable diving behaviour with maximum depths attained in excess of 1,800 m. This behaviour provides a plausible evolutionary explanation for the morphological specializations that allow M. tarapacana and potentially other large pelagic rays to tolerate cold water, and highlights potential ecological connections between surface waters and meso- and bathypelagic communities in the open ocean. Horizontal and vertical movements Chilean devil rays moved considerable distances through oligotrophic temperate, subtropical and tropical waters of the central North Atlantic Ocean. All four rays tagged in 2011 moved due south, with straight-line distances between tag deployments at Princess Alice seamount and tag pop-up locations ranging from 2,500 to 3,800 km, and average minimum swimming speeds (straight-line distance between tag deployment and pop-up locations divided by deployment duration) ranging from 24 to 44 km d −1 ( Fig. 1a ). Rays tagged in 2012 moved straight-line distances ranging from 57 to 3,182 km from the tagging location, with average minimum swimming velocities ranging between 4 and 49 km d −1 ( Fig. 1 ). 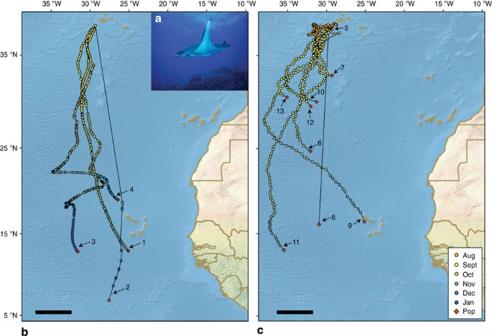Figure 1: Horizontal movements ofMobula tarapacanatagged in the Azores. (a) AdultM. tarapacanaon Princess Alice seamount where all tags were deployed. (b) Movements of individual rays (n=4) tagged in 2011 estimated from light level data recorded by pop-up satellite archival transmitting (PSAT) tags (scale bar=500 km). (c) Movements of individuals (n=9) tagged in 2012 (scale bar=500 km). Numbers next to pop-up locations reference ID numbers inTable 1andFig. 2. Basemap credits: ESRI, US National Park Service. Figure 1: Horizontal movements of Mobula tarapacana tagged in the Azores. ( a ) Adult M. tarapacana on Princess Alice seamount where all tags were deployed. ( b ) Movements of individual rays ( n =4) tagged in 2011 estimated from light level data recorded by pop-up satellite archival transmitting (PSAT) tags (scale bar=500 km). ( c ) Movements of individuals ( n =9) tagged in 2012 (scale bar=500 km). Numbers next to pop-up locations reference ID numbers in Table 1 and Fig. 2 . Basemap credits: ESRI, US National Park Service. Full size image Depth and temperature profiles collected in 2011 and 2012 revealed behaviours that differ significantly from the findings of earlier Mobula studies. Daily depth and temperature data showed that individuals tagged in 2011 dove to maximum depths ranging from 1,736 to 1,896 m with corresponding minimum water temperatures between 3.6 and 4.4 °C ( Fig. 2 ). Moreover, tagged individuals were regularly travelling to bathypelagic depths, with one individual diving below 800 m on one-third of the 80 days after tag deployment, and below 1,400 m on six consecutive days during this period ( Fig. 2a ). We observed similar deep-diving behaviour in nine rays tagged in 2012, with daily maximum depths and minimum temperatures between 416 and 1,848 m, and 4.2 and 12.8 °C, respectively. The only individuals ( n =3) that did not dive below 800 m had premature tag releases after less than 25 days of deployment ( Table 1 ). Overall, tagged rays spent an average of 4.9% of their time at mesopelagic depths (range 0–15.3%), and 0.5% of their time at bathypelagic depths (range 0–3.8%). 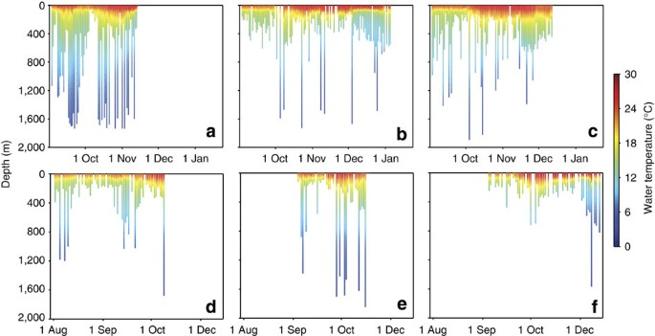Figure 2: Ambient water temperatures experienced byMobula tarapacana. Daily temperature records, as a function of depth, from the time of tag deployment until tag pop-up in the central North Atlantic Ocean, logged by the three pop-up satellite archival transmitting tags with the most complete data recovery deployed in 2011 (top panels) and 2012 (bottom panels) (a) ID=1 (b) ID=2 (c) ID=4 (d) ID=7 (e) ID=12 (f) ID=13. Figure 2: Ambient water temperatures experienced by Mobula tarapacana. Daily temperature records, as a function of depth, from the time of tag deployment until tag pop-up in the central North Atlantic Ocean, logged by the three pop-up satellite archival transmitting tags with the most complete data recovery deployed in 2011 (top panels) and 2012 (bottom panels) ( a ) ID=1 ( b ) ID=2 ( c ) ID=4 ( d ) ID=7 ( e ) ID=12 ( f ) ID=13. Full size image Table 1 Tag information for Mobula tarapacana deployments. Full size table Dive profiles We identified a total of 49 dive profiles with maximum depths of at least 800 m, beyond the vertical extent of oxygen minimum layers in the tropical and subtropical North Atlantic [12] . These dives generally followed one of two distinct patterns ( Fig. 3 ). The most common profile involved descent to the maximum depth followed by a slower, stepwise return to the surface with a total dive time of 60 to 90 min ( Fig. 4 ). Tagged rays generally only made one such dive during a 24-h period, although on two occasions an individual produced two deep dives with surface intervals of <1 h. We also identified a second dive pattern where individuals descended and then remained at depths of up to 1,000 m for as long as 11 h ( Fig. 3c ). This second profile was, however, only identified in a total of three dives. Deep dives were more frequent during the day ( n =28) than at night ( n =21), and daytime dives were longer (mean=130 min±47 s.d.) than night dives (mean=87 min±26 s.d.). Archival tags recorded the mean vertical descent velocities up to 6.0 m s −1 ( Fig. 5 ). The rays descended and ascended faster during daytime dives than at night. Descent rates on dives were faster than ascents during daytime dives; however, we found no difference between ascent and descent rates during night dives. 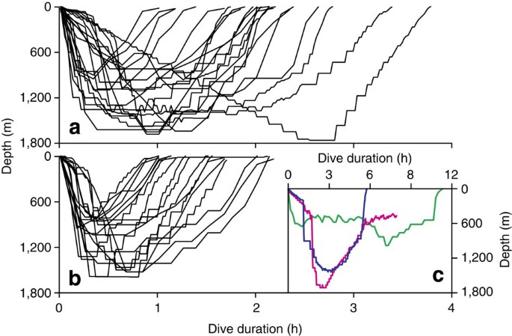Figure 3: Summary of complete dive profiles from taggedMobula tarapacana. (a) Daytime dives (n=28) of less than 4 h total duration. (b) Nighttime dives (n=21) of less than 4 h total duration. (c) Dives (n=3) with total durations longer than 4 h. Figure 3: Summary of complete dive profiles from tagged Mobula tarapacana . ( a ) Daytime dives ( n =28) of less than 4 h total duration. ( b ) Nighttime dives ( n =21) of less than 4 h total duration. 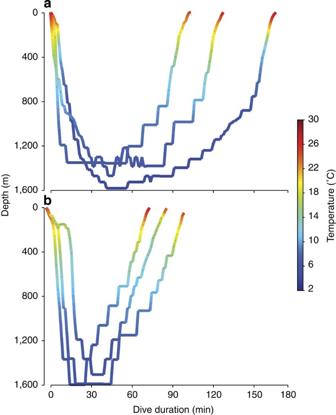Figure 4: Dive profiles from taggedMobula tarapacana. (a) Depth and temperature profiles recorded at 75 s intervals from three representative dives initiated during daylight hours (6.00 am–6.00 pm local time). (b) Depth and temperature profiles recorded at 75 s intervals from three representative dives initiated during nighttime hours (6.00 pm–6.00 am local time). ( c ) Dives ( n =3) with total durations longer than 4 h. Full size image Figure 4: Dive profiles from tagged Mobula tarapacana. ( a ) Depth and temperature profiles recorded at 75 s intervals from three representative dives initiated during daylight hours (6.00 am–6.00 pm local time). ( b ) Depth and temperature profiles recorded at 75 s intervals from three representative dives initiated during nighttime hours (6.00 pm–6.00 am local time). 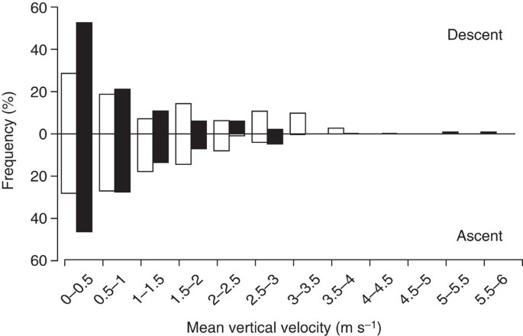Figure 5: Vertical movement rates of taggedMobula tarapacana. Frequency histograms of vertical dive rates (n=21) during descent and ascent, averaged over 75 s, from complete dive profiles initiated during daylight hours (open bars) and nighttime hours (solid bars). Full size image Figure 5: Vertical movement rates of tagged Mobula tarapacana . Frequency histograms of vertical dive rates ( n =21) during descent and ascent, averaged over 75 s, from complete dive profiles initiated during daylight hours (open bars) and nighttime hours (solid bars). Full size image Finally, we compared patterns of surface residency immediately before and after deep dives (>800 m) with all other times when the rays were not exhibiting deep-dive behaviour ( Fig. 6 ). During daylight hours, when basking at the surface would presumably result in elevated body temperatures, devil rays spent consistently more time between 0 and 2 m for up to 1 h before and 1 h after a deep dive (59% and 73% of the time, respectively) than during non-diving intervals when they were at the surface 21% of the time. 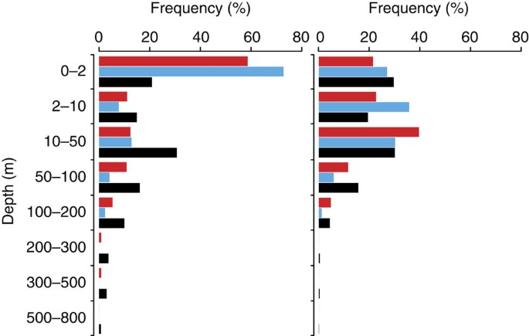Figure 6: Depth preferences ofMobula tarapacanawhile performing deep dives. (a) Daytime hours (6.00 am–6.00 pm). (b) night. Depth frequencies calculated from high resolution (75 s) depth profiles up to 1 h before (red bars,n=469 and 460 during the day and night, respectively) and after (cyan bars,n=336 and 252 during the day and night, respectively) deep (>800 m) dives, and when individuals were not diving beyond 800 m (black bars,n=90,331 and 91,336 during the day and night, respectively). However, during nighttime hours this pattern changed markedly and we found little difference in patterns of surface residency before (21.4%) or after (27%) a deep dive compared with all other times (29.6%) when the rays were not diving beyond 800 m. Figure 6: Depth preferences of Mobula tarapacana while performing deep dives. ( a ) Daytime hours (6.00 am–6.00 pm). ( b ) night. Depth frequencies calculated from high resolution (75 s) depth profiles up to 1 h before (red bars, n =469 and 460 during the day and night, respectively) and after (cyan bars, n =336 and 252 during the day and night, respectively) deep (>800 m) dives, and when individuals were not diving beyond 800 m (black bars, n =90,331 and 91,336 during the day and night, respectively). Full size image Satellite archival tagging results from the central North Atlantic revealed that M. tarapacana is a truly oceanic species capable of traversing long distances through oligotrophic tropical and subtropical waters. All tagged rays remained in oceanic environments throughout the deployments, and it is clear that M. tarapacana is capable of rapid, long-distance migrations throughout the Atlantic Ocean. Our results are in contrast with data from PSAT deployments on Mobula japonica in the eastern Pacific [10] and Mobula mobular in the Mediterranean Sea [11] . Horizontal movements by devil rays in both these studies were much more limited than those we observed. Most of the rays tagged in our study also frequently dived to depths of at least 1,500 m and were consistently encountering ambient water temperatures <5 °C. These results expand the known vertical and thermal habitat of mobulid rays by over 1,000 m and 10 °C, respectively. Tagged M. tarapacana generally moved south towards the equator from the tagging location in the Azores. Although light-based geolocation is not sufficiently accurate to determine whether the rays had travelled south together, this would appear unlikely based on both the timing and locations of the tag releases from 2011 and 2012. The rays moved at minimum speeds as high as 49 km per day between tagging and pop-up locations. These velocities are considerably faster than what has been recorded for other pelagic species including basking sharks ( Cetorhinus maximus ) [13] and whale sharks ( Rhincodon typus ) [14] that typically travel at minimum speeds of less than 30 km per day. However, a minimum speed of 112 km per day was recorded by a single female white shark ( Charcharodon charcharias ) swimming from South Africa to Western Australia [15] . While horizontal movements were not as rapid as those of the white shark, the tagged rays were capable of sustaining minimum speeds almost twice those reported for the large planktivorous sharks above. Our results revealed that M. tarapacana is among the deepest-diving ocean animals. Several marine mammal and fish species have been observed diving through the mesopelagic zone to bathypelagic depths below 1,500 m. Cuvier’s beaked whales make the deepest dives of any air-breathing animal observed to date with a maximum measured dive of 2,992 m (ref. 16 ), while a dive of 1,926 m by a whale shark currently represents the deepest published dive record for any fish species [17] . Whale sharks have also been shown to begin bathypelagic dives by descending immediately from surface waters to the deepest profile depth but then they ascend by making regular oscillations that get progressively shallower over time [18] . Tagged rays in our study, however, interspersed ascents with periods of swimming at relatively constant depths for several minutes. While a majority of these deep dives were during the day, M. tarapacana makes at least some deep forays during the night. Northern elephant seals ( Mirounga angustirostris ) [19] and Cuvier’s beaked whales [16] also dive to bathypelagic depths, presumably to forage, during both day and nighttime hours. Dive durations in the elephant seals, but not in the beaked whales, are also typically shorter during the night than during the day. The observation that both elephant seals and devil rays make shorter dives at night may be related to prey distribution as physiological constraints on diving behaviour in air-breathing elephant seals and mobulid rays are likely to be very different. It is also appears likely that the rays are raising their body temperatures before commencing a dive by basking at the surface during daylight hours, which may allow them to remain at depth for longer periods than when diving during the night. Individuals spent considerable time at the surface both immediately before and after a deep dive during the day, but not at night, suggesting that solar heating was used to raise body temperatures both before initiation of a deep dive and during dive recovery. Dive profiles for M. tarapacana exhibited descent rates of up to 6 m s −1 . By comparison, beaked whales [16] and sperm whales [20] typically dive at vertical speeds of 1–2 m s −1 , while maximum vertical dive velocities recorded for Atlantic bluefin tuna ( Thunnus thynnus ) [21] and yellowfin tuna ( T. albacares ) [22] were 4–5 m s −1 . Vertical descent rates exhibited by M. tarapacana were, then, at least as rapid as some of the ocean’s fastest swimming fishes and marine mammals. We were unable to attribute specific behaviours to M. tarapacana during dives due to limitations of the technology used. The species has been reported to prey on both pelagic crustaceans [23] and small fishes [24] . We suspect that the tagged rays were feeding on the dense layers of deep pelagic organisms that are present in the central North Atlantic [5] . Several characteristics of the most common dive profile provide strong, albeit circumstantial, evidence that the rays are indeed foraging at depth. Deep scattering layers are usually more pronounced during the daytime when many vertically migrating species are concentrated at depth [25] . These patterns are, therefore, at least consistent with the hypothesis of more, or more productive, foraging activity during daylight hours. Dive profiles of this type were characterized by rapid descents with slower ascents, a pattern also reported in several shark species and interpreted as prey-searching behaviour [26] . The step-wise ascents that we found in many of the profiles were consistent with the hypothesis that the rays were feeding on fish or squid in high-density layers at depth. Direct acoustic or visual confirmation using different technologies will, however, be needed to test this hypothesis. We also identified several long deep-dive profiles of up to 11 h during which the rays were exposed to water temperatures <10 °C for long periods. Basking sharks are the only other elasmobranch that we are aware of that performs comparably long dives to these depths and temperatures [13] . It would be difficult for the rays to maintain body heat during the long-duration deep dives and therefore these dives may be associated with travelling rather than foraging, as has been proposed for reef mantas [27] . However, additional tagging efforts are required to gain a better understating of these long dives. In such cases, it would presumably be unnecessary to maintain heightened brain function or visual acuity at depth if foraging activity during these long-duration dives was either limited or absent. Observations that individuals spend a significant amount of time at depths below 800 m and in water temperatures <10 °C provide an explanation for the enigmatic presence of retia mirabilia in the pectoral fins and cranial cavity of M. tarapacana . Pectoral muscles are the primary organ for locomotion in rays, and red muscle fibres in these fins are likely to generate significant heat that is then transferred to the brain and other sensory organs. However, it was not clear why M. tarapacana would benefit from retia that have been postulated to maintain brain function of warm-blooded sharks when foraging at depth in cold waters [28] . The dive profiles documented here show the potential benefits of a heat-exchange system that would maintain elevated cranial temperatures while foraging at depth. The presence of retia in the pectoral fins may also explain the rapid descents that we observed in the dive profiles. Active swimming by the rays would presumably produce a significant amount of heat that would then be available to warm the cranial cavity for the duration of the dive. Finally, the presence of cranial endothermy in M. tarapacana provides another line of evidence that these animals are actively foraging at depth. The energetic costs of heating the brain and sensory systems have presumably been balanced by significant foraging success during deep dives, as has been hypothesized for other fishes with cranial rete including billfishes, tunas and lamnid sharks [6] , [28] . With an estimated biomass of between 10 9 and 10 10 T wet weight, pelagic deepwater fishes represent a critical, yet understudied, component of open ocean ecosystems [1] , [29] . It has, for instance, proven particularly difficult to determine connections between predators normally observed in epipelagic habitats and the fishes, squids and octopods that together constitute the DSLs in mesopelagic and bathypelagic habitats. Vertical linkages within the open ocean are likely important to a number of commercially important fishes including bigeye tuna [30] , swordfish [3] and blue sharks [31] in the Atlantic Ocean. For instance, ommastrephid squids were the most common item in stomachs of Atlantic swordfish ( Xiphias gladius ), yellowfin tuna and albacore tuna ( Thynnus alalunga ) from the central North Atlantic, although mesopelagic fishes were also identified from samples of all three species [32] . Fatty acid profiles have provided at least some basis for speculation that whale sharks may be feeding on mesopelagic prey in the Indian Ocean [33] . Our observation that M. tarapacana frequently descended beyond depths recorded for any of these species underscores how little we know about myliobatoid rays and their potential role in open ocean food webs. This ignorance has significant conservation implications, given the large numbers of manta and devil rays either harvested to supply growing demand for their gill rakers in Asia or incidentally taken in tuna purse seine and longline fisheries [34] . More substantive efforts to monitor devil ray populations and to gain a better understanding of the ecological role that myliobatoid rays play in ocean ecosystems are, therefore, urgently needed if we are to ensure their future. Tag deployment We deployed 15 pop-up satellite archival transmitting (PSAT) tags (4 Mk-10AF and 11 MiniPAT; Wildlife Computers Inc., Redmond, WA, USA) on adult Mobula tarapacana at Princess Alice seamount, ~80 km southeast of the island of Faial in the Azores archipelago in 2011 and 2012. Deployments averaged 113 days (range 71–148 days) in 2011 and 52 days (range 13–93 days) in 2012. We programmed shorter deployments in 2012 to maximize temporal resolution of recorded dive profiles. A freediver applied PSAT tags in the dorsal musculature along the margin of the pectoral fin using a sling spear. While it is often difficult to deploy PSAT tags on large free-swimming animals, deployment lengths in our study were similar to those reported for a smaller Mobula species ( Mobula japonica ) where it was possible to capture and restrain the rays before tagging [10] . Most of the tags reported before the programmed pop-up date presumably due to problems with dart retention. Once released from the fish, the tags transmitted summarized data via the Argos satellite system until battery failure. All data from tags that released prematurely after less than 10 days were removed from all analyses. Analysis of tag data Transmitted data were decoded with manufacturer software (WC-DAP 3.0, Wildlife Computers Inc), and all subsequent analyses were conducted in the R Statistical Environment [35] . Position estimates were performed with a state-space Kalman filter model utilizing filtered sunrise and sunset times in the trackit library for R [36] . Following state-space estimation, bathymetric correction was applied using the analyzepsat library in R [37] to incorporate maximum daily depth M. tarapacana experienced. Maps were created with ArcGIS v.10.1 (ESRI Inc., Redlands, CA, USA) using a basemap created by the US National Park Service. Tags recorded light level, depth and water temperature every 5 and 10 s for the MiniPAT and Mk-10AF, respectively. These data were summarized internally for every 12-h period into 14 (MiniPAT) or 16 (Mk-10AF) temperature and depth bins. In addition, depth–temperature profiles were compiled over a 12 (Mk-10AF)- or 24 (MiniPAT)-h period, and light levels were concurrently recorded with depth to incorporate attenuation in post processing. The PSAT tags also recorded high-resolution (75–600 s) depth data from a single 48-h period every 30 days for tags deployed in 2011, and for the entire deployment period for tags from 2012. We characterized ‘deep dives’ as any profile with a maximum depth of >800 m that both initiated and terminated at depths <50 m. We only used dives with full descent and ascent profiles when calculating summary dive statistics. Ethics statement This study was performed according to national Portuguese laws for the use of vertebrates in research, and the work and tagging protocol approved by the Azorean Directorate of Sea Affairs of the Azores Autonomous region (DRAM/SRRN ref. 24/2010). How to cite this article: Thorrold, S. R. et al. Extreme diving behaviour in devil rays links surface waters and the deep ocean. Nat. Commun. 5:4274 doi: 10.1038/ncomms5274 (2014).